Carbon-catalysed reductive hydrogen atom transfer reactions Generally, transition metal catalysts are essential for the reductive hydrogen atom transfer reaction, which is also known as the transfer hydrogenation reaction or the borrowing-hydrogen reaction. It has been reported that graphene can be an active catalyst in ethylene and nitrobenzene reductions, but no report has described carbon-based materials as catalysts for alcohol amination via the borrowing-hydrogen reaction mechanism. Here we show the results from the preparation, characterization and catalytic performance investigation of carbon catalysts in transition metal-free borrowing-hydrogen reactions using alcohol amination and nitro compound/ketone reduction as model reactions. XPS, XRD, SEM, FT-IR and N 2 adsorption–desorption studies revealed that C=O group in the carbon catalysts may be a possible catalytically active site, and high surface area is important for gaining high activity. The activity of the carbon catalyst remained unchanged after reuse. This study provides an attractive and useful methodology for a wider range of applications. Hydrogen atom transfer is the most common reaction and is the fundamental step in many processes, ranging from combustion, aerobic oxidation and reduction to enzymatic catalysis and the destructive effects of reactive oxygen species [1] . In practical transformations, two types of reactions are involved in the hydrogen atom transfer reaction (that is, oxidation and reduction [2] ). In oxidation reactions, the hydrogen atom transfer initially occurs between the starting material/hydrogen donor and the catalyst, and the hydrogen atom is then removed by oxygen or other oxidants [3] . The classical reactions with this mechanism involve the oxidation of an alkane and an alcohol in the presence or absence of transition metal catalysts. The reductive hydrogen atom transfer reaction, which is also known as the transfer hydrogenation reaction or the borrowing-hydrogen reaction, is often observed in the reduction of ketones, nitro compounds and imines using isopropanol as the hydrogen donor or in the alcohol amination reaction [4] , [5] . Generally, this reaction has been observed in biotransformations [6] , and the presence of transition metals is essential to achieve this transformation [4] , [5] , [7] , [8] . Carbon materials, including amorphous carbon, ordered mesoporous carbon, graphite/graphene (oxide) and carbon nanotubes, are widely applied in many catalytic transformations in modern organic chemistry [9] , [10] , [11] , and good performance has been obtained in the oxidation of an alkane [12] , [13] , [14] , [15] , alcohol [16] , [17] , [18] , amine [19] , thiol and sulphide [20] , [21] . These reactions encompass the oxidative hydrogen atom transfer reactions. In addition, the O-rich carbon materials have been active catalysts in various reactions (that is, nucleophilic addition of alcohol to an epoxide [22] , aldehyde acetalization or esterification [23] , [24] , Michael addition reactions [25] , [26] , F-C addition of indoles to α,β-unsaturated ketones [27] and synthesis of dipyrromethane [28] , among others [29] , [30] ). In these studies, nearly all of the organic transformations have been focused on oxidative hydrogen atom transfer reactions or acid-catalysed reactions with heteroatom-modified carbon materials ( Fig. 1 ). It has been reported that graphene or phosphonium salt can be an active catalyst in olefin [31] , [32] and nitrobenzene [33] reductions, but no report has described carbon-based materials as catalysts for alcohol amination via the borrowing-hydrogen reaction mechanism. 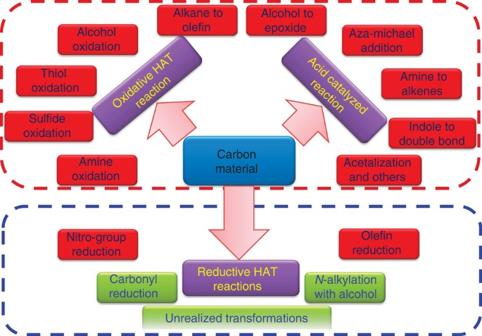Figure 1: Organic transformations catalysed by carbon materials. Carbon materials are widely applied in many catalytic transformations, including selective oxidation, nucleophilic addition and olefin/nitrobenzene reduction, but no report has described carbon-based materials as catalysts for alcohol amination via the borrowing-hydrogen reaction mechanism. Figure 1: Organic transformations catalysed by carbon materials. Carbon materials are widely applied in many catalytic transformations, including selective oxidation, nucleophilic addition and olefin/nitrobenzene reduction, but no report has described carbon-based materials as catalysts for alcohol amination via the borrowing-hydrogen reaction mechanism. Full size image In this study, we report new results on the preparation, characterization and catalytic performance of carbon materials in reductive hydrogen transfer reactions (that is, the alcohol amination reaction and ketone and nitrobenzene reduction with isopropanol as the hydrogen donor). The results suggest that the above-mentioned transformations are efficiently catalysed by carbon materials without the addition of transition metals. Catalyst preparation The carbon materials were prepared via sol-gel polymerization of resorcinol and formaldehyde with Na 2 CO 3 as a catalyst ( Fig. 2 ). First, a wet RF gel was prepared by polymerization of resorcinol and formaldehyde using a hydrothermal method. Then, the wet RF gel was mixed with KOH or another base and heated at 800 °C under a nitrogen flow. Next the carbonized sample was washed with deionized water to remove the base, and the carbon material was obtained. A series of carbon materials was prepared using this method by varying the amount and type of base. The carbon materials that were not treated with a base are denoted C-0. C-1, C-2, C-3 and C-4 were prepared using various bases (that is, KOH, NaOH, K 2 CO 3 and Na 2 CO 3 , respectively) with a fixed ratio of wet RF gel to base (that is, 1:1). Catalysts C-5, C-6 and C-7 were prepared by varying the mass ratio of the wet RF gel to KOH (that is, 1:0.25, 1:0.5 and 1:1.25, respectively). 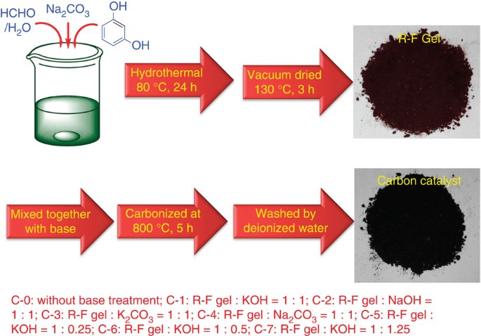Figure 2: An illustration of the carbon catalyst preparation. (1) Sol-gel polymerization of resorcinol and formaldehyde using the hydrothermal method. (2) The wet RF gel was mixed with base and heated at 800 °C under a nitrogen flow. (3) The carbonized sample was washed with deionized water to remove the base. Figure 2: An illustration of the carbon catalyst preparation. (1) Sol-gel polymerization of resorcinol and formaldehyde using the hydrothermal method. (2) The wet RF gel was mixed with base and heated at 800 °C under a nitrogen flow. (3) The carbonized sample was washed with deionized water to remove the base. Full size image Catalyst screening and optimization of the reaction conditions Alcohol amination is one of the classical reactions using the borrowing-hydrogen reaction mechanism [7] , [8] . In addition, alcohol amination is a potential approach for green and economic N -alkyl amine synthesis because alcohol is readily available, and water is generated as the sole byproduct [7] , [8] . Over the past few decades, various transition metals, such as Ru [34] , [35] , [36] , Ir [37] , [38] , Rh [39] , Pd [40] , [41] , [42] , Pt [43] , Au [41] , [44] , Ag [45] , [46] , Ni [47] , [48] , [49] , [50] , Mn [51] , [52] , Cu [53] , [54] , [55] , [56] , [57] , [58] and Fe [59] , [60] , [61] , have been employed as homogeneous or heterogeneous catalysts in the alcohol amination reaction and have yielded good results. Because it is challenging to involve the carbon catalyst in the hydride formation, carbon catalysts have not been applied to this transformation. Thus, alcohol amination was chosen as the model reaction to explore the reactivity of the carbon catalysts. The application of carbon catalysts in this reaction can offer a novel catalyst for this transformation and can aid our understanding of the hydrogen atom transfer mechanism in the absence of transition metals. The catalytic performance of the carbon materials was first explored in the benzyl alcohol amination reaction ( Table 1 ). Only 60% conversion of aniline and a 42% yield of N -benzyl aniline were obtained when C-0 was directly used as the catalyst (entry 1). Generally, the modification of the carbon material with bases, such as KOK, NaOH and K 2 CO 3 , can significantly improve the catalytic performance, and an N -benzyl aniline yield of >99% was obtained with the C-1 catalyst, which was modified with KOH (entries 2–4). In this case, there were no imines or tertiary amines observed by gas chromatography-flame ionization detector (GC-FID) and —gas chromatography–mass spectrometry. Interestingly, the modification of the carbon with Na 2 CO 3 resulted in poor activity, and the yield of N -benzyl aniline was <5% (entry 5). The influence of the amount of base on the carbon material modification was further studied by varying the mass ratio of the RF gel to KOH (that is, 1:0.25, 1:0.5 and 1:1.25). A lower activity would be obtained if the mass ratio of RF gel to KOH was <1:1. The application of additional KOH had a smaller influence on the catalytic performance of the final carbon catalyst (entries 6–8). In addition, catalyst loading was explored, and 99% N -benzyl aniline was maintained, even when 50 mg of the carbon catalyst was employed (entries 9–11). The ratio of aniline to benzyl alcohol was reduced to 1:1.2, and the yield of N -benzyl aniline was 98%. However, when the reaction was performed at 120 or 100 °C, the yield of N -benzyl aniline decreased to 89% or 21%, respectively. The amount of base added during the reaction was further optimized. Nearly no desired product was formed when no base was added, and the yield of N -benzyl aniline was only 7%, even when 30% KOH was added (entries 16 and 17). However, the yield was substantially increased to 87 and >99% when 40 and 50% KOH were added as a co-catalyst, respectively (entries 2 and 18). When other bases, including Na 2 CO 3 , NaOH, K 2 CO 3 and KO-t-Bu, were used as catalysts, different results were obtained. Yields of 68 and 89% were obtained when NaOH and KO-t-Bu were applied, respectively. In addition, the yields were <5% when Na 2 CO 3 or K 2 CO 3 was employed (entries 19–22). The difference in activity may be due to the different strengths of the bases. Finally, to exclude contributions of contaminating transition metals to the reaction, metal loadings of Pd, Ni and Cu in catalyst C-1 were investigated by ICP-AES. The results indicated that all of the metal loadings were <0.001 wt%, but no accurate results could be obtained due to the low loadings. In addition, two catalysts (that is, Ni/C-1 and Pd/C-1 containing ~0.18 wt% Ni and 0.07 wt% Pd, respectively) were prepared as control reactions. The results were even less desirable than that obtained with C-1 (entries 23 and 24, for the explanation of the results, see the discussions below). Therefore, the catalytic activity was not derived from metal contamination. When other carbon materials, such as commercially available multi-wall carbon nanotubes, graphene, graphite and activated carbon, were employed in the reaction, the results were less desirable than that obtained using C-0 as a catalyst (entries 25–29). Therefore, the catalytic activity of our catalyst is unique for the alcohol amination reactions. In addition, note that air/oxygen should be excluded because it is detrimental to borrowing-hydrogen reactions. For example, the conversions of benzyl alcohol were 75–95% with 0–14% N -benzyl aniline yields when the reactions were performed under O 2 with C-0 to C-6 as catalysts ( Supplementary Table 1 ). The major byproduct was N -benzylideneaniline. The optimized reaction conditions for benzyl alcohol amination with aniline are as follows: 1 mmol aniline, 1.2 equiv. benzyl alcohol, 50 mg catalyst, 50 mol% KOH, 2 ml toluene, Ar, 130 °C and 24 h. Table 1 Catalyst screening and optimization of the reaction conditions*. Full size table Note that the carbon catalyst can be easily recovered and reused. After the reaction, the carbon was recovered, washed with acetone, separated by centrifugation and dried for use in subsequent applications. The reaction was studied with aniline and benzyl alcohol in a molar ratio of 1:2, and the carbon catalyst exhibited stability for up to five runs without any deactivation (entry 2). Amine N -alkylation with benzyl alcohol The catalytic performance of the carbon catalyst in the alcohol amination reactions with respect to amine and alcohol derivatives was explored. First, the amination reactions of alcohol with different amines were explored ( Table 2 ). Various structurally diverse amines, regardless of the presence of electron-withdrawing or electron-donating functional groups, were monoalkylated with benzyl alcohol to yield the corresponding secondary amines in excellent yields. For example, N -benzyl aniline was synthesized in 99% yield at 130 °C (entry 1). The substituents at different positions on the aniline significantly affected the reaction rate. For example, a lower yield was obtained when o -methylaniline was used as a substrate compared with p -methylaniline and m -methylaniline (entries 2–4). The reaction tolerated the presence of halogens (entries 5–7), and 90–99% yields of the desired products were observed when o -, m - or p -chloroanilines were used as starting materials. However, the lower reaction rate of o -chloronitrobenzene relative to those of the para- and meta-analogues indicated a steric effect. The reaction of 2-aminobiphenyl and benzyl alcohol resulted in a 92% yield using a prolonged reaction time of 36 h (entry 8). Aniline derivatives, heteroaromatic amines, substituted benzyl amines, aliphatic secondary cyclic amines and aliphatic primary amines produced high yields of the corresponding secondary amines, demonstrating the high versatility of the current methodology for secondary amine synthesis (entries 9–16). Table 2 Benzyl alcohol amination with amines*. 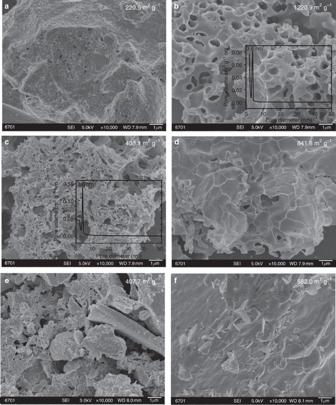Figure 3: SEM images of the carbon materials. (a) C-0, (b) C-1, (c) C-2, (d) C-3, (e) C-4 and (f) C-5 (scale bar, 1 μm). Full size table Aniline N -alkylation with alcohol derivatives The reaction also proceeded successfully with other structurally and electronically diverse alcohols ( Table 3 ). Benzyl alcohol with moderately activating groups reacted smoothly and furnished excellent yields of the respective mono- N -alkylated anilines (entries 1–6). The substituent at the ortho position had a substantial effect on the reaction. Harsher conditions (that is, higher temperatures and increased time) were required to obtain high yields when o -chlorobenzyl alcohol, o -methoxybenzyl alcohol and o -methylbenzyl alcohol were used (entries 2, 5, 8). Alcohols with a chlorine substituent reacted with aniline to afford the corresponding products with 100% conversion but with a low yield due to the dechlorination reaction (entries 7–8). Unfortunately, the reactions with a fluorine and bromine substituent were unsuccessful. Nearly no reaction was detectable and the results are not listed in the table. A prolonged reaction time of 36 h was required to produce a high yield of the desired product when p -isopropylbenzyl alcohol was used as the substrate (entry 9). The C-1 catalyst also exhibits promise for direct coupling of aniline with simple electron-poor heteroaromatic alcohols under similar conditions in moderate yields (entries 10–11, 13–14). p -Methylthiobenzyl alcohol was converted to the respective secondary amine in high yield. Unfortunately, aliphatic primary alcohols and aliphatic secondary cyclic alcohols failed to yield any product under similar conditions. Table 3 Results of the amination reaction of alcohols*. Full size table Nitrobenzene reduction with isopropanol As discussed above, in the reductive hydrogen atom transfer reactions, there are two classical reactions, that is, transfer hydrogenation of nitro compounds [62] , [63] , [64] and carbonyl group reduction [65] , [66] , [67] . In addition, it has been shown that carbon can function as an active catalyst for nitrobenzene reduction with hydrazine as the hydrogen source [33] . 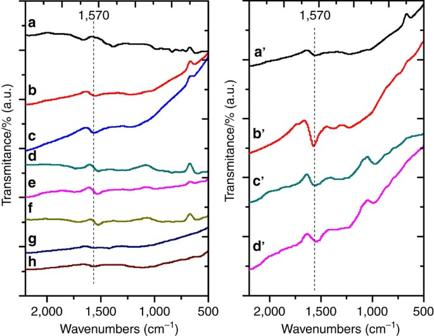Figure 4: FT-IR spectra. FT-IR spectra of C-0 to C-5 (a–f), 0.18 wt% Ni/C-1 (g), 0.07 wt% Pd/C-1 (h) and C-1 treated with oxygen and alcohol (a′: C-1;b′: C-1-O and C-1/KOH were treated with oxygen at 150 °C for 24 h;c′: C-1-O-R and C-1-O/KOH were treated with isopropanol at 150 °C for 24 h;d′: C-1-U and C-1 were reused for five runs in the coupling reaction of aniline and benzyl alcohol). Therefore, the catalytic activity of catalyst C-1 in nitro compound reductions was further tested, and the results are shown in Table 4 . For the catalytic reduction of nitrobenzene and its derivatives with a methyl group at various positions on the aromatic ring, the corresponding aniline derivatives were synthesized with up to an 88% yield (entries 1–5). The major byproducts were azobenzene and azoxybenzene, based on the gas chromatography–mass spectrometry and GC-FID analyses. On the basis of the appearance of the reaction mixture, it is possible that a small amount of high molecular weight material was formed, but this possibility was difficult to determine. The presence of other functional groups, such as acetyl, halogen and phenyl groups, only had a small influence on the reaction, and similar results were obtained with a prolonged reaction time (entries 6–9). A good yield was also obtained when 1-nitronaphthalene was employed as a starting material (entry 10). Therefore, the carbon catalyst exhibited good activity for the reduction of nitrobenzene derivatives using isopropanol as a hydrogen donor. Table 4 Reduction of nitro compounds with isopropanol as the hydrogen donor*. 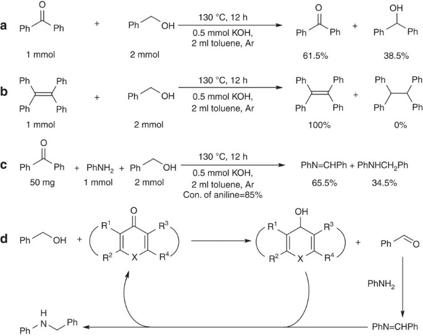Figure 5: Reaction mechanism exploration. (a) Reaction of benzophenone and benzyl alcohol; (b) Reaction of tetraphenyl ethylene with benzyl alcohol; (c) Benzophenone catalyzed benzyl alcohol amination with aniline and (d) Possible reaction mechanism. All the results were determined by gas chromatography–mass spectrometry. Con., conversion. Full size table Ketone reduction with isopropanol The catalytic reduction of ketones with isopropanol as a hydrogen donor was performed using C-1 as a catalyst, and the results are listed in Table 5 . Acetophenone derivatives containing different substituents were efficiently transformed into the corresponding alcohols in up to 99% yields (entries 1–7). Although no dechlorination reactions were observed for the reduction of p -Cl-acetophenone, debromination and dechlorination reactions occurred when 2,4-dichloroacetophenone and p -Br-acetophenone were applied as starting materials. In addition, 1-(naphthalenyl)-2-ethanone, propiophenone and benzophenone could be reduced smoothly, and the yields of the desired products were 98–99% (entries 8–10). The catalytic reduction of cyclic ketones, such as cyclohexanone and cyclooctanone, was also achieved in 91–99% yields (entries 11–13). In addition, linear ketones with different alkyl chain lengths could be used as starting materials, and these compounds afforded the desired products in 98% yields (entries 14–15). Therefore, our carbon catalyst system can be employed with ketone derivatives with versatile structures. Table 5 Ketone reduction with isopropanol as the hydrogen donor*. Full size table Catalyst structure and reaction mechanism Next the carbon catalysts were characterized by X-ray photoelectron spectroscopy (XPS), Brunauer–Emmett–Teller (BET), X-ray diffraction (XRD), scanning electron microscopy (SEM) and Fourier transform infrared spectroscopy (FT-IR) to explore the structure of the active catalyst. The C1 s spectra suggested that catalysts C-1 to C-5 possess similar surface carbon species. In addition, the O1 s spectra of the different carbon materials were different ( Supplementary Fig. 1 ). Active catalysts C-1 and C-3 exhibited a similar activity, although their O1 s spectra were different. The less active catalyst (C-4) possessed an O1 s spectrum that was similar to that of the most active catalyst (C-1). Similar phenomena were observed from the surface C:O ratios. The surface C:O ratios of C-0, C-1, C-3, C-4 and C-5 were over the range of 7:1 to 8:1. However, the surface C:O ratio of C-2 was 16:1. Therefore, it is difficult to explain the variations in catalytic activity based on the XPS characterization results. The catalysts were also characterized by XRD. Although the diffraction patterns are not shown, similar results were obtained from all of the catalysts, and nearly all of the carbon materials were amorphous. Next the carbon catalysts were characterized using s.e.m. and the nitrogen adsorption–desorption method. The SEM images of the different catalysts indicated that the treatment of the RF gel with base before carbonization resulted in the formation of a different porous structure ( Fig. 3 ). The porosity of the carbon materials was consistent with their BET surface areas. The surface area of C-0, which was not treated with a base, was only 220.5 m 2 g −1 , and the surface areas were 1,220.9, 408.1, 841.8, 407.7 and 582.0 m 2 g −1 for catalysts C-1 to C-5, respectively. In addition, mesoporous structures were observed in samples C-1 and C-2. However, the surface area contributed less to the catalytic performance because a similar activity was obtained with C-3. The high BET surface area, along with the mesoporous structure, may be responsible for the high catalytic activity. In addition, the BET surface areas of Ni/C-1 and Pd/C-1 were 1,168 and 1,268 m 2 g −1 , respectively, and may not be responsible for their relatively low activities compared with C-1. Figure 3: SEM images of the carbon materials. ( a ) C-0, ( b ) C-1, ( c ) C-2, ( d ) C-3, ( e ) C-4 and ( f ) C-5 (scale bar, 1 μm). Full size image To determine the possible active site on the carbon catalyst, FT-IR characterization was performed, and the band associated with C=C and the strongly conjugated C=O was observed [68] , [69] . Interestingly, the variations in catalytic performance were related to the density of the C=C and C=O groups at ~1,570 cm −1 in the different catalyst samples, and the strongest adsorptions were observed in samples C-1 and C-2 ( Fig. 4a–f ). It is illogical to attribute the reactivity to the C=C group because the reverse reaction, that is, alkane dehydrogenation, is less feasible. Thus, the catalytically active site might be the C=O group. For catalysts, 0.18 wt% Ni/C-1 and 0.07 wt% Pd/C-1, the FT-IR adsorption peaks at 1,570 cm −1 were weaker than those observed in the FT-IR spectra of C-1 ( Fig. 4g,h ). Thus, the lower C=O concentrations might have caused their lower activity. To clarify this result, catalyst C-1 was treated with molecular oxygen at 150 °C to verify the variation in the FT-IR spectra ( Fig. 4a′–d′ ). The C=O adsorption band increased in intensity after the treatment of C-1 with oxygen. The intensity of this band decreased again when it was further treated with isopropanol, and acetone was formed simultaneously. These results suggested that recycling of the C=O group occurred in the transfer hydrogenation reactions. The FT-IR adsorption peaks of multi-wall carbon nanotubes, graphene, graphite and activated carbon were weak at 1,570 cm −1 , which might explain their low activities ( Supplementary Fig. 2 and Table 1 , entries 25–29). It should be mentioned that a high surface area may be important to achieve high activity as well. Figure 4: FT-IR spectra. FT-IR spectra of C-0 to C-5 ( a – f ), 0.18 wt% Ni/C-1 ( g ), 0.07 wt% Pd/C-1 ( h ) and C-1 treated with oxygen and alcohol ( a ′: C-1; b ′: C-1-O and C-1/KOH were treated with oxygen at 150 °C for 24 h; c ′: C-1-O-R and C-1-O/KOH were treated with isopropanol at 150 °C for 24 h; d ′: C-1-U and C-1 were reused for five runs in the coupling reaction of aniline and benzyl alcohol). Full size image Subsequently, benzophenone and tetraphenyl ethylene were used as the model substrates to explore the potential roles of ketone and olefin in the transfer hydrogenation reaction ( Fig. 5 and Supplementary Fig. 3 ). First, the reactions of benzophenone and tetraphenyl ethylene with benzyl alcohol were performed ( a ). As expected, 38.5% of the benzophenone was converted to benzohydrol, and benzaldehyde was simultaneously generated. For the reaction of tetraphenyl ethylene and benzyl alcohol, no tetraphenyl ethane was observed ( b ). Then, the benzophenone-catalysed amination reaction of aniline and benzyl alcohol was performed ( c ). Although this catalyst is not as active as our carbon catalyst, 85% aniline conversion was obtained and the selectivity to N -benzyl aniline was 34.5%. The byproduct was N -benzylideneaniline with 65.5% selectivity. The results suggested that benzophenone was an active catalyst for the dehydrogenation of benzyl alcohol to generate benzaldehyde, but it was less active in the transfer hydrogenation of N -benzylideneaniline to produce N -benzyl aniline. Therefore, these results support the catalytic recycling between C=O and CHOH. In addition, the alcohol amination reaction of aniline with benzyl alcohol was performed with the addition of 5 mol% butylated hydroxyl toluene or 2,2,6,6-tetramethylpiperidine-1-oxyl to determine whether the reaction is radical-based (for the reaction conditions, see Table 1 , entry 2). The yields of N -benzyl aniline were 98 and 99%, which were nearly the same as the C-1/KOH catalyst system. So, the incorporation of a radical-based mechanism in the carbon-catalysed reductive hydrogen atom transfer reactions can be excluded. On the basis of these discussions, a reaction mechanism was proposed ( d ). Generally, in the alcohol amination reaction, (1) the alcohol was transformed to an aldehyde via hydrogen transfer from the alcohol to the C=O groups of the carbon catalyst; (2) the aldehyde reacted with the amine to generate an imine; and (3) the hydrogen was transferred from the carbon catalyst to the imine, resulting in the formation of an N -alkyl amine and the regeneration of the C=O group. Figure 5: Reaction mechanism exploration. ( a ) Reaction of benzophenone and benzyl alcohol; ( b ) Reaction of tetraphenyl ethylene with benzyl alcohol; ( c ) Benzophenone catalyzed benzyl alcohol amination with aniline and ( d ) Possible reaction mechanism. All the results were determined by gas chromatography–mass spectrometry. Con., conversion. Full size image In summary, the transition metal-free reductive hydrogen atom transfer transformation was realised using a carbon material as the catalyst with alcohol amination as well as nitro compound and ketone reduction as model reactions. The carbon catalyst exhibited excellent catalytic performance and good generality in the above reactions. The catalyst/product separation was easily performed, and the carbon catalyst was recyclable for several runs without observable deactivation. The results suggested that the C=O group may be the catalytically active site in this catalyst, while a high surface area of the carbon catalyst is important for achieving high activity. The activity of the base-activated carbon catalyst remained unchanged during the reuse process due to its stable structure. This new catalytic system may provide an attractive and useful methodology for a wider range of applications for industrially important compounds and intermediates. General XRD measurements were conducted on an X’Pert PRO (PANalytical) diffractometer. The XRD diffraction patterns were scanned in the 2 θ range of 10 to 80°. The XPS measurements were performed using a Thermo Scientific ESCALAB 250 instrument with a dual Mg/Al anode X-ray source, a hemispherical capacitor analyser and a 5 keV Ar + ion-gun. All of the spectra were recorded using non-monochromatic Mg Kα (1,253.6 eV) radiation. Nitrogen adsorption–desorption isotherms were measured at 77 K using a Micromeritics 2010 instrument. The pore size distribution was calculated using the Barrett, Joyner and Halenda method from the desorption isotherm. FT-IR spectroscopy characterizations were performed on a Nicolet 5700 spectrometer. The sample was prepared by mixing 0.5 mg carbon material with 100 mg KBr. SEM was performed with a JEOL JSM-6701F equipped with a cold FEG (Field Emission Gun). The metal loadings of the catalysts were measured with an inductively coupled plasma-atomic emission spectrometry (ICP-AES) instrument (ARL Co. USA, 3520). NMR spectra were measured using a Varian NMR system at 400.1 MHz ( 1 H) and 100.6 MHz ( 13 C). All spectra were recorded in CDCl 3 and chemical shifts ( δ ) are reported in p.p.m. relative to tetramethylsilane referenced to the residual solvent peaks. Typical procedure for the preparation of the carbon catalysts The carbon materials were prepared via sol-gel polymerization of resorcinol and formaldehyde with Na 2 CO 3 as a catalyst. Generally, resorcinol (R, 2.20 g, 20 mmol), formaldehyde (F, 3.25 g, 40 mmol, 36.5% in water, methanol stabilized) and 9 ml of distilled water were added into a 100- ml PTFE autoclave. Then, 22.1 mg of Na 2 CO 3 (1 mol% to resorcinol) was added to the mixture. After vigorous stirring for 1 h, the autoclave was sealed and maintained at 80 °C for 1 day. Then, the autoclave was cooled to room temperature. The wet gels were placed in a round-bottom flask and vacuum dried at 130 °C for 3 h. Next the RF gel and KOH were mixed with a mass ratio of 1:1 (1.5 g/1.5 g) and carbonized at 800 °C for 5 h under a nitrogen flow (20 ml min −1 ). The resulting carbon material was ultrasonically washed with distilled water until neutral (100 ml × 5) and dried at 80 °C for 6 h. Finally, ~730 mg of the carbon material was obtained and denoted C-1. Several carbon materials were prepared using the same procedure involving treatment of the RF gel and different bases (that is, NaOH (1.5 g/1.5 g), K 2 CO 3 (1.5 g/1.5 g) and Na 2 CO 3 (1.5 g/1.5 g)), and the resulting carbon materials are referred to as C-2, C-3 and C-4, respectively. By varying the amount of KOH (that is, 0.375 g, 0.75 g and 1.88 g), carbon materials C-5, C-6 and C-7 were obtained, respectively. For comparison, the RF gel itself was also carbonized at 800 °C for 5 h under a nitrogen flow (20 ml min −1 ), and the final sample was called C-0. C-1-O was prepared by treating C-1 (400 mg C-1, 112 mg KOH, and 4 ml toluene) under 1 MPa oxygen atmosphere at 150 °C for 24 h. C-1-O-R was obtained by treating C-1-O (400 mg C-1-O, 112 mg KOH, and 2 ml isopropanol) with isopropanol at 150 °C for 24 h. C-1-U refers to catalyst C-1 being used for five runs in the coupling reaction of aniline and benzyl alcohol, as shown in Table 1 , entry 2 and Supplementary Fig. 1 . Multi-wall carbon nanotubes (Shenzhen Nanotech Port Co., surface area: 40–300 m 2 g −1 ), graphite (Sinopharm Chemical Reagent Co.), graphene (prepared using the arc-discharge method by the Laboratory of Clean Energy Chemistry and Materials, LICP, CAS, surface area: 30–100 m 2 g −1 ), AC-Vulcan XC-72 (Vulcan XC-72 carbon, Cabot, USA, surface area: ~200 m 2 g −1 ) and AC-KB (Henan Huaxian Activated Carbon Company, surface area: ~2,000 m 2 g −1 ) were used for control reactions. Typical procedure for benzyl alcohol amination with aniline All of the reactions were performed in a pressure tube. Aniline (1 mmol), 2 mmol benzyl alcohol, 100 mg of catalyst C-1, 0.5 mmol KOH and 2 ml of toluene were added to a pressure tube followed by exchange with Ar. The tube was sealed and maintained at 130 °C for 24 h. After completion of the reaction, the tube was cooled to room temperature, and 1 mmol of biphenyl and 10 ml of EtOH were added for quantitative analysis with a GC-FID (Agilent 7890 A). The crude mixture was purified by column chromatography. The 1 H and 13 C NMR spectra and characterization data of the isolated compounds were given in Supplementary Figs 4–23 and Supplementary Methods . Typical procedure for nitrobenzene reduction All of the reactions were performed in a Shrek tube. Nitrobenzene (1 mmol), 100 mg of catalyst C-1, 3 mmol KOH and 2 ml of isopropanol were added to a Shrek tube followed by exchange with H 2 . Then, the tube was sealed and maintained under a H 2 atmosphere at 100 °C for 24 h (H 2 balloon). After completion of the reaction, the tube was cooled to room temperature, and 1 mmol of biphenyl and 10 ml of EtOH were added for quantitative analysis with a GC-FID (Agilent 7890 A). The crude mixture was purified by the following steps. First, the isopropanol was removed on a Rot-Vap. Then, the aniline was extracted by CH 2 Cl 2 , and pure aniline was obtained after removing the CH 2 Cl 2 and vacuum drying. The 1 H and 13 C NMR spectra and characterization data of the isolated compounds were given in Supplementary Figs 24–29 and Supplementary Methods . Typical procedure for acetophenone reduction All of the reactions were performed in a Shrek tube. Acetophenone (1 mmol), 100 mg of catalyst C-1, 1 mmol KOH and 2 ml of isopropanol were added to a Shrek tube followed by exchange with H 2 . Then, the tube was sealed and maintained under a H 2 atmosphere at 100 °C for 24 h (H 2 balloon). After completion of the reaction, the tube was cooled to room temperature, and 1 mmol of biphenyl and 10 ml of EtOH were added for quantitative analysis with a GC-FID (Agilent 7890 A). The crude mixture was purified by the following steps. First, the catalyst was removed by filtration. Then, the pure product was obtained after removing the organic solvent and vacuum drying. The 1 H and 13 C NMR spectra and characterization data of the isolated compounds were given in Supplementary Figs 30–34 and Supplementary Methods . How to cite this article: Yang, H. et al. Carbon-catalysed reductive hydrogen atom transfer reactions. Nat. Commun. 6:6478 doi: 10.1038/ncomms7478 (2015).